Encapsulation of single-molecule magnets in carbon nanotubes Next-generation electronic, photonic or spintronic devices will be based on nanoscale functional units, such as quantum dots, isolated spin centres or single-molecule magnets. The key challenge is the coupling of the nanoscale units to the macroscopic world, which is essential for read and write purposes. Carbon nanotubes with one macroscopic and two nanoscopic dimensions provide an excellent means to achieve this coupling. Although the dimensions of nanotube internal cavities are suitable for hosting a wide range of different molecules, to our knowledge, no examples of molecular magnets inserted in nanotubes have been reported to date. Here we report the successful encapsulation of single-molecule magnets in carbon nanotubes, yielding a new type of hybrid nanostructure that combines all the key single-molecule magnet properties of the guest molecules with the functional properties of the host nanotube. The findings may pave the way to the construction of spintronic or ultrahigh-density magnetic data storage devices. Single-molecule magnets (SMM) possess a wide range of functional properties unique to this class of materials, including magnetic bistability [1] , quantum tunnelling of magnetization [2] , [3] , and quantum coherence [4] , [5] . These properties are unattainable in other types of magnetic molecules, including endohedral fullerenes, such as N@C 60 , which, however, exhibits much longer electron spin relaxation times [6] , [7] , [8] than those of SMM. The properties of SMM can be exploited for applications in molecular electronics [9] , spintronics [10] , data storage devices [11] and quantum information processing [12] . However, any practical application of SMM requires their interaction with the macroscopic world, to allow read-and-write processes. A possible approach to this end is deposition of SMM on conductive surfaces, which, however, often leads to SMM decomposition [13] , [14] . Carbon nanotubes (NT) offer an excellent solution to connecting SMM to the outside world, without attendant problems of deterioration of the SMM functionality. The state of the SMM in such a hybrid NT–SMM material can be controlled electrically, because NT are excellent electrical conductors [14] . Such electrical control is essential for local addressability for data storage, spintronics or quantum information processing applications [15] , [16] . Furthermore, NT are chemically and thermally very robust, which is highly advantageous for device fabrication [17] . Finally, the nanotube that encapsulates the SMM also protects the guest molecule from the surroundings that would otherwise induce strong decoherence, which is highly detrimental for quantum information processing applications [18] . The magnetic bistability of SMM, essential for data storage applications, derives from a combination of two factors [11] . The intramolecular superexchange interactions give rise to a well-defined ground state with high spin. For example, the ground state of the archetypical SMM, [Mn 12 O 12 (O 2 CCH 3 ) 16 (H 2 O) 4 ] or Mn 12 Ac for short, has a spin of S =10. Secondly, the zero-field splitting parameter D is large and negative, leading to a preferential magnetization direction, the easy axis. These two factors combined result in a large energy barrier for magnetization reversal, which gives rise to slow relaxation of the magnetization and concurrent magnetic bistability. The shape of M 12 Ac can be described as a discoid with a diameter of 1.6 nm and a height of 1.1 nm ( Fig. 1a ). Considering the minimum van der Waals gap of 0.3 nm required between the surface of the molecule and the inner surface of NT [17] , the smallest diameter of NT capable of hosting Mn 12 Ac is 2.2 nm. Therefore, insertion of Mn 12 Ac, as indeed other SMM whose dimensions tend to be even larger, into single-walled carbon nanotubes (SWNT; typical diameter range 1–2 nm) is not feasible, and thus wider multiwalled carbon nanotubes (MWNT) (internal diameter range 5–50 nm) should be used as host-structures for SMM. Indeed, all previous attempts of combining SMM and SWNT resulted in composite structures where the molecules, adsorbed on the nanotube surface, were exposed to the detrimental influences of the environment (atmospheric oxygen and water, or ambient light), often leading to fast degradation of their magnetic properties [19] , [20] , [21] . 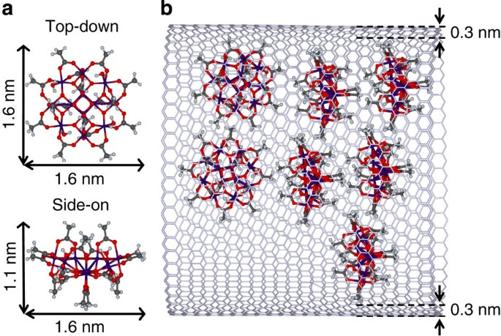Figure 1: Chemical structure of Mn12Ac SMM and schematic representation of its encapsulation in a carbon nanotube. (a) Ball and stick structure of [Mn12O12(O2CCH3)16(H2O)4] (Mn12Ac), with its dimensions indicated by double-headed arrows. Carbon, hydrogen, manganese and oxygen atoms are shown as grey, light-blue, purple and red circles, respectively. (b) Schematic representation of the innermost layer of a GMWNT hosting Mn12Ac molecules. Figure 1: Chemical structure of Mn 12 Ac SMM and schematic representation of its encapsulation in a carbon nanotube. ( a ) Ball and stick structure of [Mn 12 O 12 (O 2 CCH 3 ) 16 (H 2 O) 4 ] (Mn 12 Ac), with its dimensions indicated by double-headed arrows. Carbon, hydrogen, manganese and oxygen atoms are shown as grey, light-blue, purple and red circles, respectively. ( b ) Schematic representation of the innermost layer of a GMWNT hosting Mn 12 Ac molecules. Full size image Here we report the preparation and study of a hybrid material in which Mn 12 Ac SMM are encapsulated inside MWNT ( Fig. 1b ). We show that the SMM functional properties are fully retained, and that the molecules undergo a large degree of orientational ordering inside the nanotube. This ordering is advantageous for addressing purposes and for controlling electronic properties of the nanotube. Encapsulation of SMM into carbon nanotubes We chose graphitized MWNT (GMWNT), produced by catalytic chemical vapour deposition at 2,800 °C, with a length of 10–50 μm, and a mean internal diameter of 6.5±1.8 nm ( Supplementary Figs S1–S4 ), because these GMWNT are sufficiently wide for insertion of SMM, and are completely free of residual catalyst that complicated the analysis of the magnetic properties of other nanotube-based structures [20] . Mn 12 Ac is by far the most-studied SMM and exhibits a blocking temperature as high as 4 K, which is much higher than that of the vast majority of other SMM [11] . To allow encapsulation of Mn 12 Ac SMM, the GMWNT were pre-treated with concentrated nitric acid followed by heating in air, yielding open GMWNT with an average length of 400±200 nm. We have used supercritical CO 2 (scCO 2 ) for the transport of the SMM molecules into the nanotubes. scCO 2 is an excellent carrier fluid for the encapsulation of molecules, because the small size of CO 2 , its low viscosity, high diffusivity and zero surface tension allow it to penetrate the nanotubes without hindrance, enabling insertion of the desired guest species [22] , [23] , [24] . The mild filling conditions, with temperatures not exceeding 40 °C, allowed for the successful insertion of Mn 12 Ac, which is far too fragile to be transported into GMWNT through the gas or molten phase. The resulting hybrid material, Mn 12 Ac@GMWNT ( 1 ), was carefully washed with acetonitrile (a good solvent for Mn 12 Ac) to eliminate any Mn 12 Ac molecules outside the NT ( Supplementary Figs S5 and S6 ). The nanotubes in material Mn 12 Ac@GMWNT ( 1 ), as observed by transmission electron microscopy (TEM), comprise discrete, free-standing entities ( Fig. 2a ). There is no indication of Mn 12 Ac aggregates outside the NT in Mn 12 Ac@GMWNT, whereas in a control sample before washing ( Supplementary Fig. S7 ), these aggregates can be clearly seen. The higher magnification micrograph ( Fig. 2b ) shows a series of parallel lines corresponding to the sidewalls of the GMWNT, and dark contrast attributable to clusters of individual Mn 12 Ac molecules positioned within the GMWNT cavity ( Fig. 2d ). Indeed, energy-dispersive X-ray analysis (EDX) spectra taken from filled nanotubes using a 4 nm e-beam probe unequivocally prove the presence of manganese inside the nanotubes ( Fig. 2c ). It is noted that Mn 3 O 4 , an expected decomposition product of Mn 12 Ac, which would exhibit a characteristic crystal lattice structure in TEM, was not observed in this sample ( Supplementary Fig. S8 ), thus confirming that intact Mn 12 Ac molecules are present inside the nanotubes, consistent with the magnetic measurements described below. Under the influence of the e-beam in the TEM, the Mn 12 Ac was observed to move within the nanotube cavity ( Supplementary Fig. S9 ), indicating that the molecules are held by van der Waals forces only, with no covalent bonds formed between the SMM and the nanotube sidewalls. 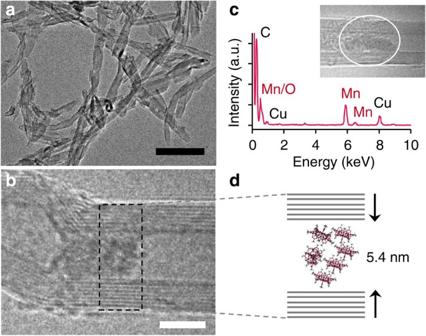Figure 2: Structural and compositional characterization of Mn12Ac@GMWNT. (a,b) Conventional bright field and phase contrast transmission electron micrographs of GMWNT filled with Mn12Ac (1) (black scale bar is 100 nm white scale bar is 5 nm). (c) EDX spectrum of the selected area in the GMWNT (inset, circled), confirming the presence of Mn-containing molecules within the nanotube (Cu peaks are due to a copper TEM support grid). (d) Schematic representation of the packing of Mn12Ac molecules in a nanotube. Figure 2: Structural and compositional characterization of Mn 12 Ac@GMWNT. ( a , b ) Conventional bright field and phase contrast transmission electron micrographs of GMWNT filled with Mn 12 Ac ( 1 ) (black scale bar is 100 nm white scale bar is 5 nm). ( c ) EDX spectrum of the selected area in the GMWNT (inset, circled), confirming the presence of Mn-containing molecules within the nanotube (Cu peaks are due to a copper TEM support grid). ( d ) Schematic representation of the packing of Mn 12 Ac molecules in a nanotube. Full size image Our encapsulation procedure combined with a washing step with acetonitrile ensures that all SMM are inside nanotubes, and that no molecules remain on the nanotube surface. A series of rigorous control experiments involving untreated (sealed) GMWNT were performed to ascertain the efficacy of the washing procedure, using exactly the same conditions as for the preparation of Mn 12 Ac@GMWNT ( 1 ) ( Supplementary Fig. S10 ). The composite of Mn 12 Ac with sealed GMWNT showed a clear signature in the powder X-ray diffractogram attributable to the presence of Mn 12 Ac clusters adsorbed on GMWNT surface, before washing ( Fig. 3a —orange). After washing, the only feature remaining in the diffractogram corresponded to the atomic lattice of sealed GMWNT ( Fig. 3a —blue). Thermogravimetric analysis (TGA) of the sealed GMWNT after washing showed that no metal-containing material remained after heating above 600 °C ( Fig. 3b —blue). Thus, both X-ray diffraction and TGA data indicate that all the Mn 12 Ac molecules have been removed from the nanotube surface in the washing step. In contrast, the hybrid material Mn 12 Ac@GMWNT ( 1 ) subjected to the same washing procedure did not lose its guest Mn 12 Ac molecules, as confirmed by TGA ( Fig. 3b —red). These experiments demonstrated that Mn 12 Ac interacts stronger with the interior of GMWNT than with its exterior because of a greater contact area of the disc-shaped molecule with the concave side as compared with the convex side of the nanotube cylinder, which ensures effective encapsulation of SMM into GMWNT driven by van de Waals force. 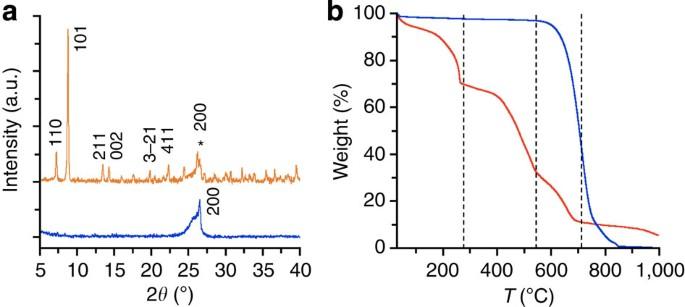Figure 3: Preferential interactions of SMM with GMWNT interior revealed through control experiments. Powder X-ray diffractograms (a) of the composite material where Mn12Ac is adsorbed on the surface of closed (untreated) GMWNT before (orange) and after (blue) washing with acetonitrile, confirming the efficient removal of Mn12Ac molecules from the nanotube surface. The peak labelled with an asterisk is assigned to the nanotube. (b) TGA of Mn12Ac@GMWNT (1) (red) and closed GMWNT after washing (blue). Figure 3: Preferential interactions of SMM with GMWNT interior revealed through control experiments. Powder X-ray diffractograms ( a ) of the composite material where Mn 12 Ac is adsorbed on the surface of closed (untreated) GMWNT before (orange) and after (blue) washing with acetonitrile, confirming the efficient removal of Mn 12 Ac molecules from the nanotube surface. The peak labelled with an asterisk is assigned to the nanotube. ( b ) TGA of Mn 12 Ac@GMWNT ( 1 ) (red) and closed GMWNT after washing (blue). Full size image The weight loss of the Mn 12 Ac@GMWNT ( 1 ) in TGA proceeded in three distinct steps ( Fig. 3b —red). The first step corresponded to decomposition of Mn 12 Ac with the loss of all coordinated ligands and, hence, the consequent formation of Mn 3 O 4 . The second step corresponded to the catalytic oxidation of the GMWNTs in the presence of the Mn 3 O 4 formed inside the nanotubes, and the third step corresponded to thermal oxidation of the GMWNT themselves (that is, sections of nanotubes that are not in direct contact with Mn 3 O 4 ) [25] , [26] . The residual weight remaining at 1,000 °C was attributed to Mn 3 O 4 that does not decompose further. The first step was also observed in the TGA of pristine, unconfined Mn 12 Ac ( Supplementary Fig. S11 ), thus supporting the fact that the Mn 12 Ac molecules remain structurally intact upon insertion into the GMWNT ( Supplementary Figs. S12–S17 ; Supplementary Tables S1–S3 ). Differential scanning calorimetry (DSC) measurements showed essentially the same Mn 12 Ac thermal behaviour before and after treatment with scCO 2 ( Supplementary Figs S12 and S13 ), again confirming that the molecules are transported and encapsulated in the GMWNT in their intact form. It is interesting to note that Mn 12 Ac molecules inside the nanotubes decompose at a slightly higher temperature ( ca. 240 °C) as compared with free molecules ( ca. 220 °C). This indicates that the confinement of SMM within the nanoscopic cavities of GMWNT enhances their thermal stability and resistance to oxidation in air. These findings demonstrate that Mn 12 Ac@GMWNT ( 1 ) fabricated in supercritical fluid is a clean, well-defined nanostructured material, with all of the SMM contained inside the nanotubes. Magnetic behaviour of SMM in nanotubes The magnetic properties of SMM inserted in nanotubes have been extensively investigated in our study ( Fig. 4 ). A control sample of free, non-encapsulated Mn 12 Ac ( 2 ), treated with scCO 2 under the same conditions as used for the preparation of Mn 12 Ac@GMWNT ( 1 ), was also studied to ascertain the influence of nanotubes on SMM properties ( Supplementary Figs S16 and S17 ). Alternating current (AC) magnetic susceptibility measurements recorded for Mn 12 Ac@GMWNT ( 1 ) ( Fig. 4a,b ) show an out-of-phase ( χ ″) signal ( Fig. 4b ) that is a manifest signature of slow relaxation of magnetization. Furthermore, both the in-phase ( χ ′) and out-of-phase ( χ ″) signals are strongly frequency dependent, indicating that the observed slow relaxation is due to the SMM behaviour, that is, the presence of an energy barrier for relaxation of the magnetic moment. It is worth noting that the observed frequency dependence of the AC signals follows an Arrhenius law, τ = τ 0 exp(Δ E / k B T ), where τ is the relaxation time of magnetization, T temperature, Δ E activation energy and k B Boltzmann constant, which allows calculation of the energy barrier (Δ E / k B ) for the relaxation process of the magnetization of molecular magnets in nanotubes ( Supplementary Fig. S19 ). Importantly, these AC magnetic susceptibility measurements confirmed that the Mn 12 Ac molecules remain intact inside the nanotube, with their functional magnetic properties fully preserved (for Mn 3 O 4, the maxima in χ ″ would occur at much higher temperatures, and would not show such a pronounced frequency dependence). To our knowledge, this is the first example of intact SMM that have been encapsulated inside nanotubes. In all previous studies, SMM mixed with SWNT were adsorbed on the external nanotube surfaces [19] , [20] , [21] . Although surface deposition of Mn 12 Ac is known to cause decomposition of the delicate magnetic molecules [13] , our procedure for the transport and encapsulation of SMM into GMWNT has no detrimental effects on the structural integrity and magnetism of the Mn 12 Ac. 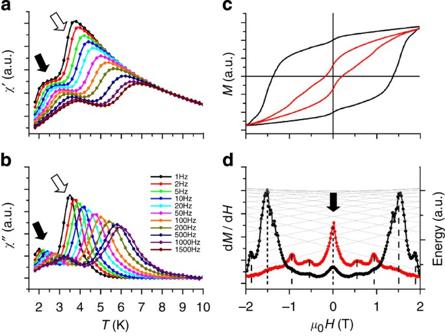Figure 4: Magnetic characterization of Mn12Ac@GMWNT. In-phase (a) and out-of-phase (b) components of the AC susceptibility of Mn12Ac@GMWNT (1) measured with an AC field of 3.5 Oe at different frequencies, showing slow relaxation of the magnetization of the encapsulated Mn12Ac molecules. (c) Hysteresis curves of magnetization recorded for Mn12Ac@GMWNT (red) at 1.8 K and for the control sample Mn12Ac (2) (black). (d) Derivatives of the hysteresis curves shown in (c), including the energy level scheme for Mn12Ac plotted as a function of field (thin crossing lines), calculated using parameters reported previously11. Figure 4: Magnetic characterization of Mn 12 Ac@GMWNT. In-phase ( a ) and out-of-phase ( b ) components of the AC susceptibility of Mn 12 Ac@GMWNT ( 1 ) measured with an AC field of 3.5 Oe at different frequencies, showing slow relaxation of the magnetization of the encapsulated Mn 12 Ac molecules. ( c ) Hysteresis curves of magnetization recorded for Mn 12 Ac@GMWNT (red) at 1.8 K and for the control sample Mn 12 Ac ( 2 ) (black). ( d ) Derivatives of the hysteresis curves shown in ( c ), including the energy level scheme for Mn 12 Ac plotted as a function of field (thin crossing lines), calculated using parameters reported previously [11] . Full size image Both χ ′ and χ ″ display two distinct maxima (labelled with arrows, Fig. 4a,b ), attributable to the presence of two slightly different Mn 12 Ac species, with different values of zero-field splitting parameter, D . The lower-temperature maximum corresponds to a fast-relaxing species in which Jahn–Teller elongation axis of one of the Mn 3+ centres has been tilted by 90° compared with the normal Mn 12 Ac molecule (slow-relaxing species) [27] . For Mn 12 Ac@GMWNT ( 1 ), the fraction of fast-relaxing species, which is determined from the intensity of the low-temperature peak, is ~20% compared with 7% for the control sample Mn 12 Ac ( 2 ) ( Supplementary Fig. S16 and Supplementary Table S4 ). This type of Jahn-Teller isomerization has also been observed previously for Mn 12 Ac aggregated in small clusters embedded in polymer matrices [28] , [29] . The SMM in nanotubes exhibit magnetic hysteresis at 1.8 K with sizeable coercivity of 0.2 T ( Fig. 4c ), again demonstrating that their properties remain largely unaffected by nanoscale confinement. Step-like features in the hysteresis curves, which become more evident in the plots of numerical derivatives d M /d H ( Fig. 4d ), are attributed to quantum tunnelling of the magnetization. The tunnelling occurs for each longitudinal field at levels ( M S states) on both sides of the magnetization relaxation energy barrier that are in resonance [2] , [3] . These steps (dotted lines, Fig. 4d ) occur at the same fields for both Mn 12 Ac@GMWNT ( 1 ) and the control sample Mn 12 Ac ( 2 ), showing both samples to have the same D values. The observed variation of the step positions with the strength of magnetic field correlates well with the crossing energy levels (thin lines, Fig. 4d ) calculated for Mn 12 Ac (ref. 11 ). These observations are consistent with a significant fraction of the molecules becoming oriented with their easy axes aligned parallel to the applied magnetic field. Without such orientation the longitudinal component of the applied field for each molecule would be different resulting in a smearing-out of the magnetization steps. The derivative peaks of the magnetization steps near zero field (labelled with a black arrow, Fig. 4d ) are due to relaxation of the fast-relaxing species, the magnetization of which is not blocked at this temperature. The relative step size found for Mn 12 Ac@GMWNT ( 1 ) is higher than for Mn 12 Ac ( 2 ), indicating more efficient quantum tunnelling and, hence, larger transverse anisotropy of the confined magnetic molecules. The lower coercitivity value in the hysteresis curve for Mn 12 Ac@GMWNT ( 1 ) ( Fig. 4c ) with respect to the control sample Mn 12 Ac ( 2 ) also confirms the shorter spin relaxation time for the confined Mn 12 Ac inside GMWNT. This observation is also in agreement with the calculated energy barrier for Mn 12 Ac@GMWNT ( 1 ) (Δ E / k B =57±1 K) that appears to be lower than for Mn 12 Ac ( 2 ) (Δ E / k B =72±4 K). Magnetoresistance of Mn 12 Ac@GMWNT Understanding the response of electric properties of Mn 12 Ac@GMWNT to applied magnetic field is crucial for future applications of this material in nano-electronic devices. The influence of a magnetic field applied parallel (θ=90°) or perpendicular (θ=0°) to a layer of Mn 12 Ac@GMWNT ( 1 ) on the resistance of the nanotubes filled with the magnetic molecules has been evaluated, and compared with a control sample of empty (short and open) GMWNT ( 3 ), the same as used for the preparation of Mn 12 Ac@GMWNT ( 1 ). Both samples Mn 12 Ac@GMWNT ( 1 ) and GMWNT ( 3 ) exhibited high room-temperature-specific conductivities of ca. 20 S cm −1 , which decrease with temperature ( Supplementary Figs S20 and S21 ) due to inter-tube contact resistance [30] , [31] . This indicates that the nanotubes filled with SMM molecules retain their intrinsic electric properties. The effect of the magnetic field on conductance of Mn 12 Ac@GMWNT became measurable only at temperatures below the blocking temperature of the single-molecule magnet Mn 12 Ac ( ca. 5 K, Supplementary Fig. S22 ) residing in nanotubes. For example, at 2 K and the field above 1 T, all samples exhibited a simple positive magnetoresistance, regardless of the direction of the applied magnetic field ( Fig. 5a ). However, at lower fields (below 1 T), the magnetoresistance of empty nanotubes and nanotubes filled with SMM are qualitatively different ( Fig. 5b ). The sample Mn 12 Ac@GMWNT ( 1 ) exhibits a significant negative magnetoresistance in this range, which is in a sharp contrast to the control sample GWMNT ( 3 ) ( Fig. 5b ; Supplementary Fig. S23 ). Another important effect of the magnetic guest molecules is that they change the response of the host nanotubes to the direction of the applied field. For example, magnetoresistance of Mn 12 Ac@GMWNT ( 1 ) becomes more negative and its minimum shifts substantially as the field changes from perpendicular ( θ =0°) to parallel ( θ =90°), whereas for empty nanotubes ( 3 ) both the depth of the minimum and its position remain unchanged. 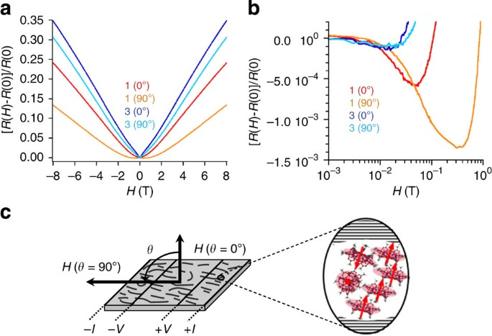Figure 5: Magnetoresistance measurements of nanotubes hosting Mn12Ac SMM. (a) Magnetoresistance of Mn12Ac@GMWNT (1) and the control sample of empty (open and short) GMWNT (3) at 2 K with magnetic field (H) either perpendicular (θ=0°) or parallel (θ=90°) to the conducting layers. (b) Low field region of the magnetoresistance measurements on the logarithmic scale. (c) Schematic representation of the device used for magnetoresistance measurements. Inset: schematic representation of the preferential alignment of Mn12Ac molecules in the internal cavity of nanotube with respect to the magnetic field. Figure 5: Magnetoresistance measurements of nanotubes hosting Mn 12 Ac SMM. ( a ) Magnetoresistance of Mn 12 Ac@GMWNT ( 1 ) and the control sample of empty (open and short) GMWNT ( 3 ) at 2 K with magnetic field (H) either perpendicular (θ=0°) or parallel (θ=90°) to the conducting layers. ( b ) Low field region of the magnetoresistance measurements on the logarithmic scale. ( c ) Schematic representation of the device used for magnetoresistance measurements. Inset: schematic representation of the preferential alignment of Mn 12 Ac molecules in the internal cavity of nanotube with respect to the magnetic field. Full size image The effects of the SMM on nanotubes can be also observed at higher magnetic field (>1 T, Fig. 5a ). The gradient of the positive magnetoresistance of Mn 12 @GMWNT ( 1 ) changes by 50% as the directions of the field changes, whereas the control sample of GMWNT ( 3 ) is significantly less sensitive showing only 10% change. Encapsulated SMM modify the susceptibility of the resistance of nanotubes to the angle of the magnetic field, which relates to a preferential orientation of the Mn 12 Ac molecules in the internal cavities of the nanotubes ( Fig. 5c ). As the Mn 12 Ac have a shape of a disc, with the easy magnetic axis perpendicular to the disc, this magnetic anisotropy of the guest molecules translates into the anisotropic magnetoresistance behaviour of the host nanotubes. This study describes a methodology for integration of SMM into the internal cavity of carbon nanotubes. The non-covalent interactions, which are responsible for efficient transport and encapsulation of the guest molecules into nanotubes, allow the molecules to stay mobile within the nanotube and align along the applied magnetic field. Although the encapsulated Mn 12 Ac molecules retain their SMM properties, the host nanotubes provide an alternative pathway for relaxation of SMM magnetization. In turn, the magnetic guest molecules influence the electrical resistance of the host nanotubes. Therefore, the new class of hybrid structures SMM@GMWNT represents a synergistic material combining the functional properties of nanotubes and magnetic molecules. Encapsulation of SMM into carbon nanotubes offers a number of exciting opportunities for the applications of these materials in nano-electronics. For example, electrical conductivity of the nanotube that could be precisely controlled by the magnetic states of SMMs can provide a method for generating spin-polarized currents at the nanoscale, which are important for the emerging area of spintronic devices. Insertion of SMMs into carbon nanotubes may enable integration of these molecular materials into ultrasensitive magnetic devices, such as a nanoscale superconducting quantum interference device (nano-SQUID) or a magnetic force microscopy probe, which will open a pathway for harnessing functional properties of SMMs at a single-molecule level—a long-standing challenge in molecular nanomagnetism [32] . Preparation of materials Mn 12 Ac was synthesized following the procedure described previously [33] . All reagents and solvents were purchased from Sigma-Aldrich and used without further purification. GMWNT (catalysed chemical vapour deposition) were purchased from CheapTubes. GMWNT were pre-treated to shorten and open them, and to enable the encapsulation of Mn 12 Ac molecules. Preparation of short and open GMWNT via oxidative cutting GMWNT (200 mg) were added to a 16 M solution of nitric acid (50 ml) and the resulting black suspension was treated with ultrasound in a water bath for 30 min at room temperature. The suspension was then heated in air under reflux for 5 h. The resulting mixture was then diluted with deionized water (200 ml), filtered using a 0.45 μm pore size PTFE membrane filter, washed thoroughly with water until neutral pH and ethanol (50 ml) and dried under vacuum to yield a black solid (192 mg). The product was then placed in an alumina crucible and heated in air at 700 °C until weight loss of 80% was achieved. Encapsulation of Mn 12 Ac in GMWNT Freshly annealed GMWNT (10 mg, short and open) were added to a suspension of Mn 12 Ac (30 mg) in hexane (8 ml), and the resulting black suspension was transferred into a 10 ml autoclave that was topped up with supercritical carbon dioxide (40 °C, 275 bar). The pressure was cycled between 270 bar and 120 bar for 20 h. The resulting black solid was then washed with 250 ml acetonitrile and filtered using 0.2 μm pore size PTFE membrane filter to give Mn 12 Ac@GMWNT ( 1 ). Control measurements A series of rigorous control experiments involving untreated (sealed) GMWNT were performed to ascertain the efficacy of the washing procedure, and therefore, less effective interactions of Mn 12 Ac molecules with the outer surface of the nanotubes as compared with the interior of GMWNT ( Supplementary Figs S7 and S10 ). To confirm that Mn 12 Ac molecules are transported and encapsulated in the GMWNT in their intact form, a control sample of Mn 12 Ac ( 2 ) treated with scCO 2 under the same conditions as used for preparation of 1 was carefully analysed by different analytical techniques all supporting the fact that structure and properties of Mn 12 Ac remain unchanged ( Supplementary Figs S11–S17 and Supplementary Tables S1–S3 ). To prove that the Mn 12 Ac remains intact inside NT, the thermal properties of Mn 12 Ac@GMWNT ( 1 ) were characterized by DSC and TGA. Additionally, a Mn 12 Ac@GMWNT sample heated at 340 °C was analysed by TEM ( Supplementary Figs S24 and S25 ), revealing that Mn 3 O 4 is formed as a product of thermal decomposition of Mn 12 Ac in GMWNT. To verify that Mn-peaks in the EDX are indeed due to Mn 12 Ac guest molecules, EDX spectra were taken for empty sections of nanotubes in Mn 12 Ac@GMWNT and the supporting carbon film, none of which showed any indication of Mn ( Supplementary Fig. S26 ). Analytical techniques TGA measurements were carried out on a SDT Q-600 TA instrument over the range 25–1,000 °C in air and at a scan rate of 5 °C min −1 . DSC measurements were carried out on a Mettler Toledo DSC 821e over the range 25–500 °C with a scan rate of 5 °C min −1 in air or nitrogen. X-ray powder diffraction measurements were performed on a PANalytical X'Pert PRO diffractometer equipped with a Cu Kα radiation source (λ=1.5418 Å) in Bragg–Brentano geometry using a Si zero-background holder. Infrared spectra were measured as KBr discs on a Nicolet Avatar 380 FTIR spectrometer over the range 400−4,000 cm −1 . Elemental analyses were performed by the Elemental Analysis Service of London Metropolitan University. Mass spectrometry was carried out on a Bruker ApexIV with electro spray ionization. Transmission electron microscopy characterization High-resolution TEM imaging and energy-disperse X-ray analyses were performed using a Jeol 2100F transmission electron microscope using an accelerating voltage of 100 kV. TEM samples were prepared by casting several drops of hexane suspension of Mn 12 Ac@GMWNT onto copper-grid mounted 'lacey' carbon films before drying under a stream of nitrogen. Statistical analysis of TEM images were performed using Gatan Digital Micrograph software. Magnetic measurements A commercial Quantum Design MPMS-XL5 SQUID magnetometer was used for the magnetic characterization of the samples: Mn 12 Ac@GMWNT ( 1 ), Mn 12 Ac (post-scCO 2 ) ( 2 ) and pristine Mn 12 Ac. Pellet samples were pressed and wrapped into Teflon film with negligible diamagnetic contribution. Variable-temperature (1.8–300 K) and field-dependent (0–5 T) magnetization measurements were carried out using the reciprocating sample option with a sensitivity of 5×10 −9 emu. AC susceptibility measurements were carried out at different frequencies (1–1,500 Hz) of a 3.5 Oe oscillating field between 1.8 and 10 K. Methodology used in the magnetic measurements The investigation of the effects of the encapsulation into nanotube on the magnetic properties of Mn 12 Ac molecules was carried out by comparing the results obtained for 1 with those for 2 and untreated Mn 12 Ac taking into account the diamagnetic contribution of GMWNT. Considerations in the magnetic analysis of 1 The analysis of the magnetic measurements of 1 requires the quantification of both the diamagnetic contribution of the GMWNT and the molar concentration of Mn 12 Ac in the sample. To disentangle the effects of the GMWNT on the magnetic properties of the Mn 12 Ac molecules, we first measured the magnetic response of the empty GMWNT. The magnetization loop ( Supplementary Fig. S27 ) shows that GMWNT do not exhibit hysteresis. Moreover, GMWNT have diamagnetic response, because the measured magnetization is negative for positive fields and positive for negative fields. The linear response of M versus μ 0 H allows the determination of the susceptibility χ =(−10.0±0.1)×10 −8 emu cm −3 that is simply given by the slope of the curve. The susceptibility measurements for GMWNT as function of the temperature are presented in Supplementary Figure S28 . The signal from the GMWNT is always negative, that is, diamagnetic (of the order of −6.38×10 −6 emu g −1 at 300 K) and slightly increases below 42 K (inset Supplementary Fig. S28 ). The mass susceptibility of Mn 12 Ac is 2.83×10 −5 emu g −1 at 300 K that is 77% higher than that of the GMWNT. Below 100 K the difference in mass susceptibility increases further with the Mn 12 Ac reaching 9.03×10 −3 emu g −1 at 1.8 K that is three orders of magnitude higher than that of the GMWNT at the same temperature. The quantification of the molar concentration has been carefully assessed from the magnetic measurements reported in Supplementary Figure S27 . M GMWNT , M Mn12Ac and M Mn12Ac@GMWNT were defined as the magnetic moments of the GMWNT, Mn 12 Ac and Mn 12 Ac@GMWNT samples, respectively. If m GMWNT , m Mn12Ac and m Mn12Ac@GMWNT are their respective masses, then the magnetic moments per mass of the GMWNT and Mn 12 Ac, and , respectively, can be calculated. As m Mn12@GMWNT = m GMWNT + m Mn12Ac , the following relation holds Then the mass of Mn 12 Ac and GMWNT can be calculated as From the magnetic moment measured at 1.8 K and 2 T ( Supplementary Fig. S27 ), it can be deduced that , and M Mn12Ac@GMWNT =0.172±0.005 emu. Because m Mn12Ac@GMWNT =33.8±0.1 mg, then, m GMWNT =29.0 and m Mn12Ac =4.8±0.7 mg. Magnetoresistance measurements DC conductivity measurements were performed with the four contacts method for two pressed pellets of each sample: Mn 12 Ac@GMWNT ( 1 ) and GMWNT ( 3 ). Both pellets of each sample gave very similar results demonstrating reproducibility of the measurements. The magnetoresistance measurements were performed in the temperature range 2–300 K with magnetic fields in the range −8 to 8 T applied either parallel or perpendicular to the conduction planes. Platinum electrodes (25 μm diameter) were connected to the samples using graphite paste. The samples were measured with cooling and warming rates of 1 K min −1 and with DC intensity currents of 0.1–1.000 μA in a Quantum Design PPMS-9, giving reproducible results in all cases. Further details of the magnetoresistance measurements can be found in the Supplementary Figs S20–S23 . Quantification of the amount of SMM inside nanotubes The amount of Mn 12 Ac in Mn 12 Ac@GMWNT ( 1 ) can be estimated from TGA (11.6% wt). From the TGA measurements, the amount of Mn 12 Ac has been deducted by comparing the amount of manganese oxide remaining at 1,000 °C after all carbon of Mn 12 Ac@GMWNT being burnt out (5.6% of the total weight, Supplementary Fig. S25 ) with the residual manganese oxide found at the same temperature for pristine Mn 12 Ac (47.2% of the total weight, Supplementary Fig. S11 ). Magnetic measurements described above gave 14.2% wt for Mn 12 Ac in Mn 12 Ac@GMWNT that is slightly higher than TGA. The accuracy of quantitative SQUID measurements is expected to be greater than that of TGA. How to cite this article: Giménez-López, M.C. et al . Encapsulation of single-molecule magnets in carbon nanotubes. Nat. Commun. 2:407 doi: 10.1038/ncomms1415 (2011).